High-mobility and low-power thin-film transistors based on multilayer MoS2crystals Unlike graphene, the existence of bandgaps (1–2 eV) in the layered semiconductor molybdenum disulphide, combined with mobility enhancement by dielectric engineering, offers an attractive possibility of using single-layer molybdenum disulphide field-effect transistors in low-power switching devices. However, the complicated process of fabricating single-layer molybdenum disulphide with an additional high- k dielectric layer may significantly limit its compatibility with commercial fabrication. Here we show the first comprehensive investigation of process-friendly multilayer molybdenum disulphide field-effect transistors to demonstrate a compelling case for their applications in thin-film transistors. Our multilayer molybdenum disulphide field-effect transistors exhibited high mobilities (>100 cm 2 V −1 s −1 ), near-ideal subthreshold swings (~70 mV per decade) and robust current saturation over a large voltage window. With simulations based on Shockley's long-channel transistor model and calculations of scattering mechanisms, these results provide potentially important implications in the fabrication of high-resolution large-area displays and further scientific investigation of various physical properties expected in other layered semiconductors. The discovery of graphene opened the door to the exotic electronic, optical and mechanical properties of two-dimensional (2D) crystals [1] . Graphene has a conical Dirac spectrum of energy states without a bandgap and a linear dispersion. While these properties are the root of much of the novel electronic and optical phenomena of graphene, the gapless bandstructure also makes it unsuitable for conventional transistors for electronic switching. Similar to the storyline of the graphite and graphene family, transition metal dichalcogenides of the form MX 2 where M=metal and X=S, Se or Te are emerging as highly attractive candidates for the study of fundamental physics in 2D and in layered (thin-film) structures. These materials form layered structures, where layers of covalently bonded X–M–X atoms are held together by Van der Waals interactions. But, because of the broken symmetry in the atomic basis, they can have bandgaps of ~1 eV. Among these layered semiconductors, recently, special emphasis has been given to single-layer (SL) MoS 2 owing to its intriguing electrical and optical properties. While bulk MoS 2 is usually an n -type semiconductor with an indirect bandgap (~1.3 eV) [2] and carrier mobility in the 50–200 cm 2 V −1 s −1 range at room temperature [3] , SL MoS 2 is found [4] to have a direct bandgap of ~1.8 eV. Field-effect transistors (FETs) using SL MoS 2 exhibited high on/off ratios (~10 8 ) and low subthreshold swing (SS, ~70 mV per decade) [5] . The electron mobility of SL MoS 2 FETs varied from ~1 cm 2 V −1 s −1 (in air/MoS 2 /SiO 2 structures) to ~200 cm 2 V −1 s −1 (in HfO 2 /MoS 2 /SiO 2 structures) depending on dielectric environment. Thus, in addition to fundamental scientific interest, SL MoS 2 FETs can be an attractive alternative for electronic switches in the form of thin-film transistors (TFTs) for high-resolution liquid crystal displays and organic light-emitting diode (OLED) displays. These devices have a critical need for high field-effect mobility (>30 cm 2 V −1 s −1 ), high on/off ratio (>10 3 ), steep-subthreshold slopes for low power consumption, and electrical and optical reliabilities [6] . But, the synthesis of SL MoS 2 followed by a deposition of an additional high- k dielectric layer may not be well suited for commercial fabrication processes. Based on the physics of MoS 2 , we identify a number of reasons why multilayer MoS 2 can be more attractive for TFT application than SL MoS 2 . The density of states of multilayer MoS 2 is three times that of SL MoS 2 , which will lead to considerably high drive currents in the ballistic limit. In long-channel TFTs, multiple conducting channels can be created by field effect in multilayer MoS 2 for boosting the current drive of TFTs, similar to silicon-on-insulator MOSFETs. However, multilayer MoS 2 and corresponding dichalcogenide semiconductors have not been extensively studied for use in electronics. The characteristics in the few early reports [7] , [8] are not vastly competitive with current TFT technologies. Therefore, in this work, we explore the case of multilayer MoS 2 FETs further and show that it offers a compelling case for applications in TFTs. We report the first demonstration of multilayer MoS 2 FETs with single back-gated insulator of 50-nm-thick Al 2 O 3 by atomic layer deposition (ALD) achieving high room-temperature mobilites (>100 cm 2 V −1 s −1 ) and very low SS (~70 mV per decade), which suggest that, with a proper use of a dielectric substrate, the mobility and the SS in multilayer MoS 2 FETs may reach near the intrinsic limits at room temperature. We also demonstrate robust current saturation over a large voltage window. This is an important step towards real applications as TFTs in OLED displays are operated in the saturation region of drain current. Such saturation is elusive in FETs based on nanomaterials owing to poor electrostatic control, or exists in a very small voltage window in graphene owing to the lack of a bandgap [9] . We describe the experimental results with comprehensive simulations based on Shockley's long-channel transistor model and calculations of scattering mechanisms, and further suggest future directions to improve mobility in layered semiconductors. Device fabrication TFTs based on multilayer MoS 2 were fabricated with the architecture shown in Fig. 1a . After multilayer MoS 2 flakes were mechanically exfoliated from bulk MoS 2 crystals and transferred on ALD-Al 2 O 3 -covered Si substrates, electrical contacts of Au/Ti were patterned on top of MoS 2 flakes as described in the Methods section. Optical micrograph of a completed device is shown is Fig. 1b . The thickness of MoS 2 channels measured by atomic force microscope (AFM) was in the range of 20–80 nm. Between the two stacking polytypes that are observed in bulk MoS 2 crystals (hexagonal 2H and rhombohedral 3R) [10] , crystal orientation mapping by electron backscatter diffraction indicated only 2H MoS 2 within the measured devices as shown in Fig. 1c . Subsequent inverse pole figure in Fig. 1c confirmed that the MoS 2 channels are ‹0001›-oriented single crystals. Raman spectra of MoS 2 channels were almost identical with those of bulk single crystals as shown in Fig. 1d , and no noticeable difference in Raman shifts of MoS 2 channels were found among measured devices, indicating minimal structural modifications. 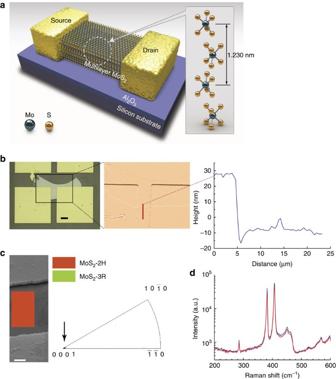Figure 1: MoS2TFT device and its structural properties. (a) Schematic perspective view of a MoS2TFT with a multilayer MoS2crystal. (b) Optical and AFM image of a device deposited on top of a silicon substrate with a 50-nm-thick Al2O3layer. The scale bar is 20 μm. Also shown is a cross-sectional plot along the red line in AFM image. (c) Scanning electron microscope image of the MoS2channel with a crystal orientation mapping. The scale bar is 3 μm. Also displayed is a partial inverse pole figure indicating a ‹0001›-oriented single crystal. (d) Raman spectroscopy measurements on a bulk single crystal (blue) and a transistor channel (red). Figure 1: MoS 2 TFT device and its structural properties. ( a ) Schematic perspective view of a MoS 2 TFT with a multilayer MoS 2 crystal. ( b ) Optical and AFM image of a device deposited on top of a silicon substrate with a 50-nm-thick Al 2 O 3 layer. The scale bar is 20 μm. Also shown is a cross-sectional plot along the red line in AFM image. ( c ) Scanning electron microscope image of the MoS 2 channel with a crystal orientation mapping. The scale bar is 3 μm. Also displayed is a partial inverse pole figure indicating a ‹0001›-oriented single crystal. ( d ) Raman spectroscopy measurements on a bulk single crystal (blue) and a transistor channel (red). 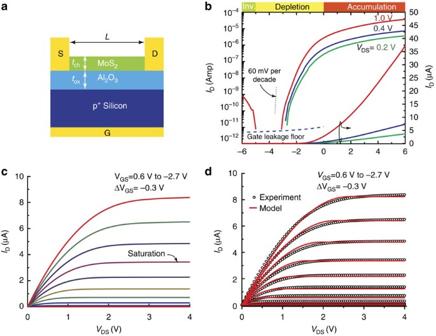Figure 2: Device geometry and electronic properties of MoS2TFTs. (a) The device geometry of a back-gated MoS2TFT. The TFT device was measured atT=300 K. The device geometries are:W/L=4/7 μm,tox=50 nm andtch=30 nm. (b) Drain current versus back gate bias showing ~106on/off ratio and ~80 mV per decade subthreshold slope. (c) Drain current versus drain bias showing current saturation. (d) Same as (c), including a long-channel model (red lines) showing excellent agreement between the TFT model and measured device behaviour. Full size image Electronic properties Figure 2 shows the measured device characteristics of a multilayer MoS 2 TFT. The thickness of the MoS 2 layer is t ch ~30 nm, and the back gate oxide thickness is t ox ~50 nm ( Fig. 2a ). Figure 2b shows the major features observed: the n -type nature of the MoS 2 layer as indicated by it turning on at positive gate biases owing to accumulation of electrons, and a window of gate biases where the device stays off (depletion). This feature was observed in all measured devices, but a fraction of the devices also showed a recovery of the current at large negative gate biases as in Fig. 2b , which is a clear indication of an inversion channel. The inversion layer formation is described further in Supplementary Fig. S4 and in the Supplementary methods . We note that the gate capacitance in this geometry is ~20 times higher than a recent report [7] . As a result, while exhibiting the high on/off ratio expected of a semiconductor with a bandgap of 1.3 eV, a sharp SS (~80 mV per decade for Fig. 2 , 70 mV per decade for some devices) is also measured at room temperature in deep depletion. In a typical field-effect geometry, the subthreshold slope is given by [11] , where C S is the capacitance in the MoS 2 conducting channel, C it = qD it is the capacitance owing to interface traps of density D it and C ox = ε ox / t ox is the oxide capacitance. Based on this model, ( C S + C it )~ C ox /3. As the semiconductor capacitance is negligible in the deep-subthreshold region, the interface trap density is D it ~2.6×10 11 eV −1 cm −2 , a very low value indeed [12] . The SS value was measured to be ~24 mV per decade at 77 K, indicating D it does not vary with temperature. We note that similar to the recent report [5] for monolayer MoS 2 , the subthreshold slope (and D it ) of multilayer MoS 2 TFTs is also exceptionally low, comparable to state-of-the-art silicon transistors. But it is obtained without the decades of processing improvement that was necessary to reduce interface trap densities between the dielectric insulator and silicon. Currently III–V semiconductors are facing the same challenge [13] . This is because of the layered nature of the semiconductor—for 2D crystals and their stacks, there are no out-of-plane broken bonds, and thus the interface traps are expected to be in the dielectrics and materials placed in contact with them, not in the semiconductor itself. This is a major advantage of MoS 2 for TFT applications. Figure 2: Device geometry and electronic properties of MoS 2 TFTs. ( a ) The device geometry of a back-gated MoS 2 TFT. The TFT device was measured at T =300 K. The device geometries are: W / L =4/7 μm, t ox =50 nm and t ch =30 nm. ( b ) Drain current versus back gate bias showing ~10 6 on/off ratio and ~80 mV per decade subthreshold slope. ( c ) Drain current versus drain bias showing current saturation. ( d ) Same as ( c ), including a long-channel model (red lines) showing excellent agreement between the TFT model and measured device behaviour. Full size image Current saturation The second major boost is seen in Fig. 2c . The drain current is observed to saturate at high drain biases for all gate voltages. The saturation occurs over a wide drain voltage window (unlike graphene). This is the first observation of a robust current saturation in a layered semiconductor composed of 2D crystals. Current saturation in transistors is an important feature towards real applications as the TFTs in OLED displays are operated in the saturation region. Like in a long-channel transistor made of a covalent semiconductor, the saturation of current occurs in the MoS 2 TFT owing to pinch-off of the conducting channel at the drain side as the gate-drain diode becomes reverse-biased at high V DS . As graphene has zero bandgap, instead of pinch-off, the drain side of the conducting channel becomes p-type at high drain bias [9] , restricting current saturation and current modulation to a very small window, if at all. The bandgap of MoS 2 makes both current modulation and saturation robust, as borne out by Fig. 2b,c . The saturation of current observed here is quantitatively understood based on a long-channel device model based on surface potential. Poisson equation is solved to determine the surface potential at the MoS 2 /ALD oxide interface as a function of the gate and the drain bias voltages. Then, the Shockley model of transistor performance is used to calculate the current. The only unknown input parameters to the model are the carrier mobility, the doping density and the contact resistance. At high positive gate biases, the channel is flooded with accumulated carriers and is highly conductive, and the contact resistances limit the current. This helps us to deduce the contact resistance to be ~17 kΩ as described in Supplementary Fig. S1 and in the Supplementary methods . This value is rather high, and reducing it by an order of magnitude is necessary for the future. Thus, the mobility and the doping density remain as the unknown parameters. In Fig. 2d , using a mobility of 100 cm 2 V −1 s −1 and a doping density of N D ~10 16 cm −3 , an excellent fit to the measured device characteristics is obtained. We assert that these values are not fortuitous, as borne out by complementary capacitance-voltage and field-effect mobility measurements, which are described next. The device model for TFTs provides insight into the performance of 2D layered semiconductor devices, and thus is a powerful tool to extract physical parameters of the material. Accumulation and inversion channels At large negative gate biases, the drain current recovers as seen in Fig. 2b , indicating the formation of an inversion channel (formation of a hole gas in a n -type semiconductor). However, the source/drain contacts are formed to the conduction band, and therefore there exists a large barrier for conduction through a p-type inversion channel. To explore these features quantitatively, capacitance-voltage measurements were performed, and the measured device characteristics were compared with energy-band diagram-based models. 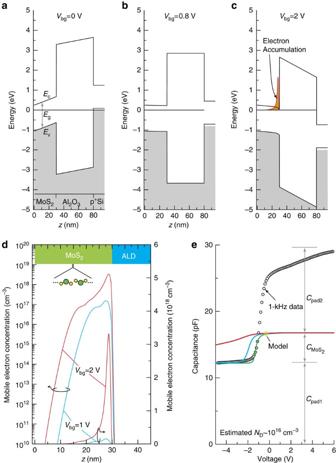Figure 3: Energy band diagrams, carrier distributions and measured capacitance-voltage profile of the MoS2TFT device. (a–c) Energy band diagrams of the MoS2/Al2O3/p+Si device under various bias conditions. The band offsets and physical parameters relevant for the calculation are described in theSupplementary methods. The self-consistent Schrödinger-Poisson calculation shows that at large positive gate bias, a 2D electron gas is formed at the MoS2/Al2O3interface. (d) The 2D electron gas that forms the conductive channel is shown in an enlarged scale. Most conduction occurs by electrons accumulated in a few layers at the MoS2/Al2O3interface. With increasing bias, the centroid of the electron distribution shifts closer to the interface. This indicates that the 'quantum' capacitance in the semiconductor increases with positive gate bias. (e) Measured capacitance-voltage curves of the MoS2/Al2O3/back-gate capacitors (circles). The solid lines show the calculated capacitance for three different doping densities (red: 1018, blue: 1017and green: 1016cm−3), not including parasitic pad capacitances. The slope indicates a doping density close to 1016cm−3. Figure 3a–c show the calculated energy band diagrams for the MoS 2 TFT structure for various gate bias conditions. For the calculation, we self-consistently solve Poisson and Schrödinger equations in the effective-mass approximation. The bandgap of SL MoS 2 occurs at the K -points in the hexagonal k-space lattice [4] , implying a valley degeneracy of g v =2, similar to graphene. On the other hand, the conduction band minimum of multilayer MoS 2 moves to a lower symmetry point in the k -space along the Γ–K line. This results in a higher valley degeneracy ( g v =6 for the Γ–K line) than SL MoS 2 , effectively tripling the density of states, implying higher carrier densities and higher currents in the ballistic limit [14] . The net drive current for a given voltage is a product of the carrier density and the velocity. Thus, in addition to high velocity, a high density of states (DOS) is equally attractive for attaining high speed. Driven by higher valley degeneracy, multilayer MoS 2 has the potential for considerably higher current drives than SL MoS 2 in the ultrascaled limit, and high charge densities have recently been reported [15] . Even in the long-channel structure, thin-film MoS 2 can take advantage of its multilayer nature. It can provide multiple conducting channels for boosting the current drive by using double gates, similar to silicon-on-insulator MOSFETs. The semiconducting material properties of multilayer MoS 2 such as the conduction and valence band offsets with Si and ALD Al 2 O 3 , the valley degeneracy, band-edge effective masses, dielectric constant and bandgap were used in the calculation. The values are provided in Supplementary Table S1 and Fig. S6 . The model indicates that owing to the work-function difference between MoS 2 and p + Si, the thin MoS 2 layer is initially depleted of mobile carriers. Upon application of positive bias on the Si gate, a 2D electron gas in the MoS 2 layers closest to the ALD Al 2 O 3 forms. This accumulation channel conducts current between the source and the drain. Figure 3d shows the accumulation carrier density profile in more detail. Most of the carriers are electrostatically confined close to the MoS 2 /ALD interface, similar to the case in a Si MOSFET. Thus, the 'quantum capacitance', which dictates the voltage drop in the semiconductor to sustain the conducting charge C S ~ ε S /‹ z › is large as the centroid of the charge distribution ‹ z › is ~1–2 nm from the interface. Figure 3: Energy band diagrams, carrier distributions and measured capacitance-voltage profile of the MoS 2 TFT device. ( a–c ) Energy band diagrams of the MoS 2 /Al 2 O 3 /p + Si device under various bias conditions. The band offsets and physical parameters relevant for the calculation are described in the Supplementary methods . The self-consistent Schrödinger-Poisson calculation shows that at large positive gate bias, a 2D electron gas is formed at the MoS 2 /Al 2 O 3 interface. ( d ) The 2D electron gas that forms the conductive channel is shown in an enlarged scale. Most conduction occurs by electrons accumulated in a few layers at the MoS 2 /Al 2 O 3 interface. With increasing bias, the centroid of the electron distribution shifts closer to the interface. This indicates that the 'quantum' capacitance in the semiconductor increases with positive gate bias. ( e ) Measured capacitance-voltage curves of the MoS 2 /Al 2 O 3 /back-gate capacitors (circles). The solid lines show the calculated capacitance for three different doping densities (red: 10 18 , blue: 10 17 and green: 10 16 cm −3 ), not including parasitic pad capacitances. The slope indicates a doping density close to 10 16 cm −3 . Full size image Capacitance measurements Figure 3e shows the measured two-terminal capacitance as a function of the voltage between an ohmic contact pad to the MoS 2 and the back gate. Several interesting features are evident from the measurement. As the pads are large as seen in Fig. 1b , they form a parasitic pad capacitance, which sets the floor of the measured value (~12 pF). When the MoS 2 layer is depleted of mobile carriers, the measured capacitance is this pad capacitance. As positive gate biases are applied, the formation of an electron accumulation layer in the MoS 2 results in an increase in the capacitance. The electron accumulation layer also electrically connects the two ohmic pads, effectively doubling the parasitic pad capacitance—this is exactly what is measured. In Supplementary Fig. S2 and the Supplementary methods , we describe this effect in more detail, and also include the capacitance-voltage measurements of a MoS 2 flake in contact with just one metal pad in Supplementary Fig. S3 , which confirms the above analysis. The capacitance of the MoS 2 layer alone ( C MML:MoS 2 ) is dependent on its doping density. The calculated values of C MML:MoS 2 for three different doping densities are shown in Fig. 3e , from which it is concluded that the unintentional doping density in the measured MoS 2 layer is of the order of N D ~10 16 cm −3 . We note that this is a low doping level, and can vary between naturally occurring samples not grown by controlled means. The extracted doping density has a direct impact on impurity scattering and carrier mobility, which is what was investigated next. Charge transport and scattering The field-effect mobility of MoS 2 TFTs was extracted from the I D - V GS curves of Fig. 2b , and the corresponding measurements for temperatures 77–300 K. The mobility values are extracted in the linear region at V GS =2 V or equivalently at a carrier density n = C ox ( V GS −V T )≈1.6×10 12 cm −2 . The intrinsic carrier mobility (mobility without the effect of the contact resistance R c ) was calculated using an equivalent circuit as shown in Fig. 4c and described further in Supplementary Fig. S5 and the Supplementary methods , and are shown as blank circles in Fig. 4a . Also shown are data reported from Fivaz and Mooser's work [3] from 1967. The values are very similar. We note here that Fivaz and Mooser used MoS 2 crystals grown by transport reaction as opposed to the naturally occurring MoS 2 used in this work, which bodes well for large-area growth for practical TFT applications. The decrease in mobility with temperature is a typical signature of diffusive band transport, as opposed to activated (hopping) transport. If there were significant Schottky barrier heights, the mobility would appear to increase with temperature. This can lead to erroneous conclusions on the nature of charge transport (that is, activated versus band transport). To avoid such confusion, samples that exhibited ohmic contacts over the entire temperature range were carefully chosen for mobility extraction. 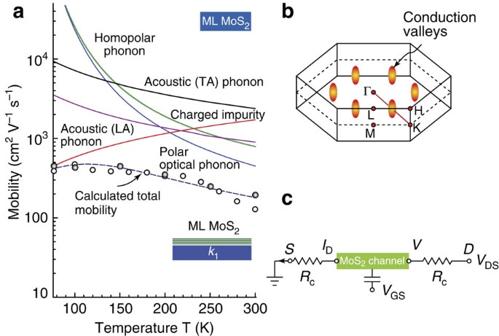Figure 4: Charge transport properties of the multilayer MoS2channel. (a) Measured temperature-dependent field-effect mobility of MoS2TFTs. The open circles are data measured in this work, and the filled circles are data from ref.3. From the theoretical transport model, the electron mobility (dashed line) is limited by impurity scattering (red line) at low temperatures. At room temperature, the mobility is limited by the combined effect of the homopolar (out-of-plane) phonon (green line) and the polar-optical phonon (blue) scattering. Details of these scattering mechanisms are described in theSupplementary methods. (b) The hexagonal Brillioun zone of multilayer MoS2with the high symmetry points and six equivalent conduction valleys. (c) An equivalent circuit model for the MoS2TFT including the effect of the contact resistanceRc. Figure 4: Charge transport properties of the multilayer MoS 2 channel. ( a ) Measured temperature-dependent field-effect mobility of MoS 2 TFTs. The open circles are data measured in this work, and the filled circles are data from ref. 3 . From the theoretical transport model, the electron mobility (dashed line) is limited by impurity scattering (red line) at low temperatures. At room temperature, the mobility is limited by the combined effect of the homopolar (out-of-plane) phonon (green line) and the polar-optical phonon (blue) scattering. Details of these scattering mechanisms are described in the Supplementary methods . ( b ) The hexagonal Brillioun zone of multilayer MoS 2 with the high symmetry points and six equivalent conduction valleys. ( c ) An equivalent circuit model for the MoS 2 TFT including the effect of the contact resistance R c . Full size image To explain the temperature-dependent carrier mobility, the semiclassical Boltzmann transport equation under the relaxation time approximation is used. The model is described in detail in the Supplementary methods . A typical characteristic of layered structures (such as MoS 2 ) is that the carriers move independently in each layer. Neglecting the vanishing interlayer interaction, the energy dispersion of carriers becomes [16] , where k =( k x , k y ) is the 2D wave vector of carriers and m * is the in-plane effective mass. The corresponding 2D density of states is , where ħ is the reduced Planck constant and g v is the valley degeneracy. Recent experiments and models indicate the conduction band minima to be along the Γ-K line [17] of the Brillouin zone, as indicated in Fig. 4b . The sixfold symmetry of this point leads to a valley degeneracy of g v =6. We have used this value for transport calculations, consistent with the energy band diagram and capacitance calculations of Fig. 3 . Carrier scattering from (a) ionized impurities, (b) acoustic phonons, (c) in-plane polar optical phonons and (d) out-of-plane lattice vibrations (homopolar phonons) are taken into account to explain the transport measurements. A 2D ionized impurity scattering model is invoked where carriers scatter from a sheet of impurities located at the surface of the MoS 2 layers. Coupling of carrier with both longitudinal acoustic (LA) phonons and transverse acoustic (TA) phonons are taken into account under the deformation potential approximation. The energies of optical phonons in bulk MoS 2 are in the frequency range of 400–500 cm −1 (50–60 meV) [19] as also measured in Fig. 1d . Electron-polar optical phonon scattering is described by the Fröhlich interaction [20] with a static dielectric constant ε 0 =7.6 and optical dielectric constant [21] ε ∞ =7.0 with phonon energy ħω op =49 meV for the E 1 2 g mode. For homopolar phonon modes, the sulphur atoms of opposite planes vibrate out of phase ( A 1 g mode) and the corresponding phonon energy is [19] , [22] ħω hp =52 meV. The resultant mobility is calculated using Mathiessen's rule . The calculated mobility associated with the individual scattering mechanisms as well as the resultant mobility is shown in Fig. 4a along with the measured data. At low temperatures, the mobility is limited by ionized impurity scattering. At room temperature, the mobility decreases by enhanced optical phonon and acoustic phonon scattering. A reasonably good match is found between calculated and experimentally measured mobility (at low temperatures) for a choice of impurity sheet density n imp ~1.8×10 10 cm −2 , which corresponds to a volume density of ~3×10 15 cm −3 . This value is comparable to the background doping density for unintentionally doped bulk MoS 2 , and consistent with the value estimated from the capacitance-voltage measurements in Fig. 3e . A large electron effective mass and the strong optical phonon (out-of-plane and polar phonon) scattering set an upper bound on the mobility in multilayer MoS 2 . We note here that the accuracy of the calculation is subject to the uncertainty in the electron–phonon coupling coefficients and the bandstructure parameters used in the model. However, these parameters are not expected to be vastly different from those assumed. Higher mobilities could potentially be achieved by intercalation of MoS 2 layers (similar to recently demonstrated encapsulations of silicon carbide crystals in graphite enclosure [23] ). By sandwiching SL MoS 2 between two dielectric layers, the out-of-plane phonon vibrations can be suppressed. If the homopolar phonon mode is damped, ionized impurity scattering and in-plane polar optical phonon scattering determine the charge transport. Strain effects can also potentially be used to deform the bandstructure, leading to lowering of the electron effective mass and improvement in mobility. Electron mobility in MoS 2 can be further expected to improve as the growth and processing methods improve, leading to fewer impurities. Moreover, charged impurity scattering in these devices can be damped using high k dielectrics (dielectric engineering) [24] , [25] , [26] . Effects such as remote phonon scattering could limit this improvement [27] . As the current experimental values are far below limits expected of remote phonon scattering, there is ample room for improvement. The mobility measured for multilayer MoS 2 already exceeds most competing semiconductor materials for large-area TFTs by orders of magnitude. The values may be further improved by proper dielectric choices to near the intrinsic phonon limits. When combined with the large current modulation, the low subthreshold slope, and robust current saturation, multilayer MoS 2 makes a compelling case for TFT applications. All these properties are achieved in a back-gated structure, without the need for an additional dielectric layer on top, which is highly attractive for TFT implementation. The first demonstration of these attractive properties, combined with the comprehensive modelling of the behaviour, is expected to move multilayer MoS 2 towards real applications. The multilayer structure is easier to achieve over large areas by chemical vapour deposition or allied techniques, which are well suited for large-area applications. Looking beyond MoS 2 , other transition metal dichalcogenides can offer competitive or complementary features. In addition to technological applications, conduction band electron states in these layered semiconductors have contributions from d orbitals, quite unlike traditional group-IV and III–V semiconductors and carbon nanomaterials, where chemical bonding is restricted to s and p orbitals. Thus, a rich range of physical phenomena that depend on d orbitals, such as magnetism, correlated-electron effects and superconductivity, can be expected in these materials. Such features can possibly be integrated with the semiconducting properties demonstrated here seamlessly, as there are no out-of-plane bonds to be broken. Device fabrication An amorphous Al 2 O 3 dielectric layer of ~50 nm in thickness was deposited on a highly doped p-type Si wafer (resistivity <5×10 −3 Ω cm) by ALD process using trimethylaluminum (TMA, UP Chemical Co. Ltd., South Korea) and H 2 O as a precursor and a reactant, respectively. The deposition temperature was maintained at 300 °C and the gas injection schedule for one cycle of deposition were 0.5/10/1.5/15 seconds for the TMA/N 2 /H 2 O/N 2 gases. Multilayer MoS 2 flakes were mechanically exfoliated from bulk MoS 2 crystals (SPI Supplies, USA) and transferred on the substrate. Electrical contacts (100 μm×100 μm) were patterned on top of MoS 2 flakes using conventional lift-off technique. Ti (10 nm) and Au (300 nm) were deposited by electron-beam evaporation at room temperature. The device was then annealed at 200 °C in a vacuum tube furnace for 2 h (100 sccm Ar and 10 sccm H 2 ) to remove resist residue and to decrease contact resistance. Measurements The thickness of MoS 2 was measured using an AFM (Nanoscope III, Digital Instruments-Veeco, USA). The electron backscatter diffraction (JEOL JSM7000F, Japan) and Raman spectra (Renishaw RM-1000 inVia, UK) with a 514-nm Ar laser were measured to characterize the MoS 2 flakes on the substrate. Electrical characterizations were carried out with current-voltage measurements (Keithley, Semiconductor Characterization System 4200-SCS). During the low-temperature measurement of transport properties, temperature was controlled using a variable temperature cryogenic probe system (LakeShore, TTPX). Capacitance-voltage characteristics were measured with an HP 4284A Precision LCR Metre. How to cite this article: Kim, S. et al . High-mobility and low-power thin-film transistors based on multilayer MoS 2 crystals. Nat. Commun. 3:1011 doi: 10.1038/ncomms2018 (2012).